Local translation ofTC10is required for membrane expansion during axon outgrowth The surface of developing axons expands in a process mediated by the exocyst complex. The spatio-temporal regulation of the exocyst is only partially understood. Here we report that stimulated membrane enlargement in dorsal root ganglion (DRG) axons is triggered by intra-axonal synthesis of TC10, a small GTPase required for exocyst function. Induced membrane expansion and axon outgrowth are inhibited after axon-specific knockdown of TC10 mRNA. To determine the relationship of intra-axonal TC10 synthesis with the previously described stimulus-induced translation of the cytoskeletal regulator Par3, we investigate the signalling pathways controlling their local translation in response to NGF. Phosphoinositide 3-kinase (PI3K)-dependent activation of the Rheb-mTOR pathway triggers the simultaneous local synthesis of TC10 and Par3. These results reveal the importance of local translation in the control of membrane dynamics and demonstrate that localized, mTOR-dependent protein synthesis triggers the simultaneous activation of parallel pathways. During the development of the nervous system, axons are guided by extracellular factors that cause rapid changes in growth cone orientation and axonal growth rates. Axon growth requires the continuous addition of new membrane to cover the greatly expanding neuronal surface. The bulk of the phospholipids forming the nascent axonal membrane is synthesized in the cell body and transported in plasma membrane precursor vesicles (PPVs) to the axonal growth cone [1] , [2] . Within growth cones, PPVs are inserted into the plasma membrane by exocytosis [3] . During the first step of this process, vesicles attach to the sites of exocytosis marked by the presence of specific effector complexes at the membrane [2] . One of these effectors is the exocyst, an evolutionarily conserved octameric protein complex comprisingSec3, Sec5, Exoc3/Sec6, Sec8, Sec10, Sec15, Exo70 and Exo84 (ref. 3) [3] , that tethers vesicles to the membrane, followed by fusion of the vesicle with the membrane leading to expansion of the plasma membrane. Currently, it is only incompletely understood how the localization and function of the exocyst is restricted to areas of membrane expansion such as growth cones. The small cdc42-like GTPase TC10 (alternative name: RhoQ) is described to control the stimulus-dependent translocation of Exoc3, Sec8 and Exo70 to the plasma membrane [4] , [5] . Thus, the current model is that TC10 activation stimulates the assembly of the exocyst leading to the tethering and secretion of PPVs at secretion sites at the membrane. This model is supported by the findings that complex formation between TC10 and Exo70 modulates neurite outgrowth in PC12 cells [6] and is essential for membrane expansion and axonal specification in developing hippocampal neurons [7] . Further, TC10 overexpression in rodent sensory neurons increases axon growth rates indicating the importance of the exocyst beyond the process of axon formation [8] . Previously, TC10 and Exoc3 mRNAs have been found in the transcriptomes of uninjured or regenerating axons, respectively [9] , suggesting that their local translation could be part of the mechanisms controlling exocyst-dependent membrane expansion. Local mRNA translation has emerged as a crucial component of the molecular pathways governing the underlying cytoskeletal changes during axon growth and guidance [10] , [11] , [12] , [13] , [14] , but the relevance of local protein synthesis for other aspects of axonal growth such as membrane expansion remains entirely unknown. Conceivably, local translation of TC10 and Exoc3 might lead to the spatially restricted formation and function of the exocyst and thus be required for membrane expansion during axon outgrowth. In addition, the coordinated local synthesis of exocyst proteins and cytoskeletal regulators such as Par3 (ref. 14) [14] might ensure that stimulus-induced cell surface expansion and cytoskeletal growth are tightly synchronized to support axon outgrowth. Here, we investigate whether local translation of TC10 or Exoc3 is required for NGF-induced axon growth and membrane expansion. We find that TC10 mRNA is localized to developing axons of DRG neurons and that its local translation is triggered by NGF and required for PPV exocytosis to the membrane during stimulated axon outgrowth. In addition, we find that inhibition of PI3K, Rheb or mTOR prevents local translation of both TC10 and Par3 mRNA, establishing an example of proteins whose coregulated local synthesis triggers the coordinated action of two parallel pathways in response to an extracellular stimulus. Membrane is added in growth cones during axon outgrowth Axons display two distinct modes of growth: basal growth in the absence of attractive stimuli is independent of local translation, while the rapid axonal elongation in response to outgrowth promoting factors requires intra-axonal protein synthesis [14] . We first investigated whether the expansion of the axonal plasma membrane during rapid outgrowth occurs within growth cones. For this we triggered axon outgrowth and hence membrane expansion in DRG neurons using nerve growth factor (NGF) stimulation. While best known as the prototypical neurotrophin, NGF is also required for the growth and targeting of sensory neuron axons during development [15] , and acts as an attractive stimulus for axons of DRG neurons [16] . Application of NGF to DRGs leads to a robust increase in axonal growth rates [14] , [17] . Thus, we cultured embryonic day 15 (E15) DRG explants and kept the neurons for 24 h before the experiment at a low NGF concentration (5 ng ml −1 ) that does not induce axon outgrowth but supports survival [14] , and triggered axonal elongation of the sensitized axons by applying a higher concentration of NGF (100 ng ml −1 ) for 1 h. Before the NGF stimulation, we applied the sphingomyelin and glucosylceramide precursor BODIPY FL C 5 -ceramide to the neurons. At high concentrations, BODIPY FL C 5 -ceramide forms excimers with an emission maximum of 620 nm but fluoresces green (515 nm) at lower concentrations [18] . This unique property causes intense red labelling of the trans-Golgi network and of Golgi-derived vesicles including PPVs in cells treated with BODIPY FL C 5 -ceramide [18] . Upon fusion of PPVs with the plasma membrane, the BODIPY label rapidly dissipates in the membrane causing the dissociation of the excimers resulting in decreased fluorescence intensity at 620 nM. The development of red labelling requires incorporation of the BODIPY-linked lipids at high concentrations in the Golgi apparatus. Many Golgi markers are present and the secretory pathway is functional in axons [19] , and axons exhibit lipid biosynthesis activity [20] , [21] . To investigate whether the red label seen in axons represented cell body-derived vesicles or originated from axonally incorporated BODIPY FL C 5 -ceramide, we used compartmentalized chambers that allow the fluidic isolation of axons from their cell bodies [22] ( Fig. 1a ) and applied BODIPY FL C 5 -ceramide only to axons. In contrast to BODIPY FL C 5 -ceramide applied to cell bodies, axonal application did not result in red labelling ( Fig. 1b ), indicating that axons are unable to incorporate the labelled sphingomyelin and glucosylceramide precursor at the required high concentration to form red fluorescent excimers. Any red vesicles seen in axons and growth cones represent, therefore, anterogradely transported Golgi-derived vesicles and are not the result of local BODIPY-ceramide metabolism or recycling of BODIPY-labelled lipids from the axonal membrane. The disappearance of red labelling from axons and growth cones is thus a direct measure of exocytosis and membrane expansion [23] . Consistent with previous reports [23] , treatment of sensitized DRGs with NGF for 1 h significantly reduced the level of red fluorescence in growth cones ( Fig. 2a ), indicating increased fusion of PPVs with the axonal plasma membrane within growth cones during stimulated axonal elongation. 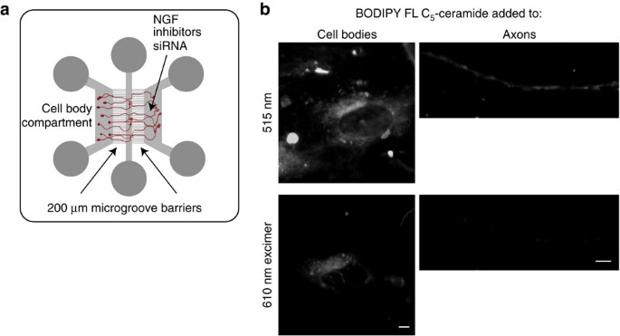Figure 1: Compartmentalized culture of DRG neurons. (a) Schematic drawing of a microfluidic chamber. Neurons are seeded into the cell body compartment. Axons have to cross two 200-μm-long microgroove barriers and a central compartment (100 μm) to reach the axonal compartment. The combination of two microgroove barriers ensures total fluidic isolation of the axonal and cell boy compartments. All agents and treatments are applied selectively to the distal axons only. (b) Application of BODIPY FL C5-ceramide to the cell body but not the axonal compartment results in intense red labelling. BODIPY FL C5-ceramide stains the cell membrane green in both compartments. Scale bars, 10 μm. Figure 1: Compartmentalized culture of DRG neurons. ( a ) Schematic drawing of a microfluidic chamber. Neurons are seeded into the cell body compartment. Axons have to cross two 200-μm-long microgroove barriers and a central compartment (100 μm) to reach the axonal compartment. The combination of two microgroove barriers ensures total fluidic isolation of the axonal and cell boy compartments. All agents and treatments are applied selectively to the distal axons only. ( b ) Application of BODIPY FL C 5 -ceramide to the cell body but not the axonal compartment results in intense red labelling. BODIPY FL C 5 -ceramide stains the cell membrane green in both compartments. Scale bars, 10 μm. 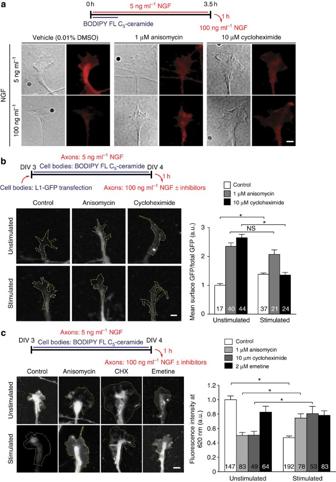Figure 2: Intra-axonal protein synthesis is required for membrane exocytosis. (a) DRG explants were incubated with BODIPY FL C5-ceramide (5 μM) and then exposed to NGF (100 ng ml−1) in the presence or absence of anisomycin (1 μM) or cycloheximide (10 μM). Cumulative fluorescence intensity was measured in growth cones and normalized to growth cone area. NGF stimulation triggered exocytosis as indicated by a decrease in the fluorescence intensity of the BODIPY label at 620 nM. Anisomycin or cycloheximide inhibited the increase in NGF-induced exocytosis. (b) DRG explants were transfected with plasmids encoding the cell adhesion molecule L1 fused to GFP. Surface GFP-L1 was measured by live staining DRG cultures with antibodies to GFP after treatment with vehicle or NGF. Treatment of axons with NGF for 1 h caused a significant increase in surface GFP in growth cones, indicating induction of exocytosis. The NGF-induced GFP-L1 translocation to the surface was sensitive to the presence of protein synthesis inhibitors. Data are mean±s.e.m. of the surface GFP fluorescence normalized to total GFP intensities of individual growth cones from three independent experiments per condition,nvalues listed represent the number of growth cones. *P<0.05 (one-way ANOVA). (c) Only the cell bodies of DRG neurons cultured in microfluidic chambers were exposed to BODIPY FL C5-ceramide for 24 h. Stimulation of axons with NGF resulted in exocytosis that was blocked by local application of anisomycin, cycloheximide or emetine. Data are mean±s.e.m. of the fluorescence intensities of individual growth cones from three independent experiments per condition,nvalues listed represent the number of growth cones. *P<0.05 (one-way ANOVA). Scale bars, 5 μm. Full size image Figure 2: Intra-axonal protein synthesis is required for membrane exocytosis. ( a ) DRG explants were incubated with BODIPY FL C 5 -ceramide (5 μM) and then exposed to NGF (100 ng ml −1 ) in the presence or absence of anisomycin (1 μM) or cycloheximide (10 μM). Cumulative fluorescence intensity was measured in growth cones and normalized to growth cone area. NGF stimulation triggered exocytosis as indicated by a decrease in the fluorescence intensity of the BODIPY label at 620 nM. Anisomycin or cycloheximide inhibited the increase in NGF-induced exocytosis. ( b ) DRG explants were transfected with plasmids encoding the cell adhesion molecule L1 fused to GFP. Surface GFP-L1 was measured by live staining DRG cultures with antibodies to GFP after treatment with vehicle or NGF. Treatment of axons with NGF for 1 h caused a significant increase in surface GFP in growth cones, indicating induction of exocytosis. The NGF-induced GFP-L1 translocation to the surface was sensitive to the presence of protein synthesis inhibitors. Data are mean±s.e.m. of the surface GFP fluorescence normalized to total GFP intensities of individual growth cones from three independent experiments per condition, n values listed represent the number of growth cones. * P <0.05 (one-way ANOVA). ( c ) Only the cell bodies of DRG neurons cultured in microfluidic chambers were exposed to BODIPY FL C 5 -ceramide for 24 h. Stimulation of axons with NGF resulted in exocytosis that was blocked by local application of anisomycin, cycloheximide or emetine. Data are mean±s.e.m. of the fluorescence intensities of individual growth cones from three independent experiments per condition, n values listed represent the number of growth cones. * P <0.05 (one-way ANOVA). Scale bars, 5 μm. Full size image Stimulated membrane expansion requires local translation To investigate whether the addition of phospholipids to the plasma membrane during axon outgrowth requires protein synthesis, we added two protein synthesis inhibitors, anisomycin and cycloheximide, to the neurons just before the stimulation with NGF. The presence of either inhibitor prevented the dissipation of the red BODIPY label, demonstrating that protein synthesis is required for membrane expansion during stimulated axon growth ( Fig. 2a ). To validate this finding with an independent approach, we used overexpressed full-length mouse L1 fused at its N terminus to GFP. The type I transmembrane protein L1 is secreted through exocytosis [3] and increased expression of GFP-L1 on the cell surface can serve as a measure for plasma membrane addition [7] , [24] . We observed dynamic changes in GFP-L1 translocation to the surface of growth cones by immunostaining living, non-permeabilized neurons with an anti-GFP antibody. Stimulation of sensitized DRG explants with NGF as before led to a significant increase in surface-exposed GFP-L1 within growth cones that was inhibited or even reversed in the presence of protein synthesis inhibitors ( Fig. 2b ). The short duration of this experiment and the fact that membrane expansion is a local process within growth cones suggested that the required protein(s) are synthesized intra-axonally, rather than in the cell body followed by anterograde transport into growth cones. To directly test this hypothesis, we added BODIPY FL C 5 -ceramide only to the cell body compartment of microfluidic chambers and sensitized the axons by lowering the NGF concentration in the side compartments as before. Stimulation of axon outgrowth by addition of NGF specifically to distal axons and growth cones induced membrane expansion as detected by the dissipation of the red label ( Fig. 2c ). Importantly, the presence of either protein synthesis inhibitor in the axonal compartment completely abolished the effect of NGF on BODIPY labelling providing evidence that local, intra-axonal translation is required for membrane expansion. In both the GFP-L1 and the BODIPY-ceramide exocytosis assays we observed a significant effect of anisomycin or cycloheximide in the absence of NGF stimulation. This might be due to side effects of the used inhibitors. For example, both anisomycin and cycloheximide activate the p38 pathway [25] , and that depending on the cellular context can have an impact on endocytic trafficking [26] or stimulate exocytosis [27] . Thus, we repeated the BODIPY-ceramide exocytosis assay using another protein synthesis inhibitor, emetine [28] , that has no effect on MAPK pathways [25] . Presence of emetine in the axonal compartment did not significantly decrease the red label under control conditions and prevented its dissipation in response to NGF stimulation ( Fig. 2c ). Endocytosis is independent of protein synthesis The increased extracellular labelling for GFP-L1 under baseline conditions in the presence of anisomycin or cycloheximide could indicate increased exocytosis or decreased endocytosis upon inhibition of intra-axonal translation as discussed above. To test the latter possibility, we performed an endocytosis assay using the fixable membrane probe FM1-43FX [29] . Uptake of FM1-43FX into distal axons and growth cones by endocytosis was monitored over 20 min in the presence or absence of protein synthesis inhibitors ( Fig. 3 ). Anisomycin or cycloheximide did not change FM1-43FX uptake rates, indicating that endocytosis is independent of local translation and that the effects seen before on GFP-L1 expression and BODIPY-ceramide excimer formation are not due to changed endocytosis rates but presumably a consequence of increased exocytosis. Together our results show that NGF-induced exocytosis is prevented in the presence of three protein synthesis inhibitors, indicating that local translation is required for NGF-induced membrane expansion. 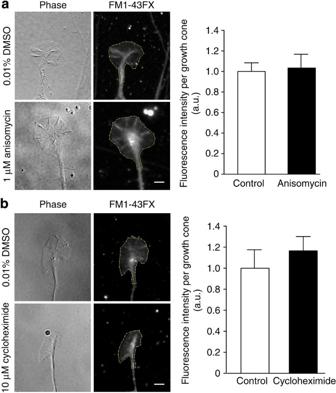Figure 3: Endocytosis does not require local translation. Axons of DRG neurons grown in microfluidic chambers were exposed to FM1-43X (10 μM) for 20 min in the presence or absence of the protein synthesis inhibitors anisomycin (a) or cycloheximide (b). Neither inhibitor affected endocytosis of the dye. Scale bar, 5 μm. Figure 3: Endocytosis does not require local translation. Axons of DRG neurons grown in microfluidic chambers were exposed to FM1-43X (10 μM) for 20 min in the presence or absence of the protein synthesis inhibitors anisomycin ( a ) or cycloheximide ( b ). Neither inhibitor affected endocytosis of the dye. Scale bar, 5 μm. Full size image TC10 is localized to axons and translated in response to NGF Next we asked which mRNA(s) that encode proteins required for membrane expansion were locally translated in response to NGF stimulation. Previously, two transcripts, Exoc3 and TC10 , coding for components of the exocyst or exocyst complex-associated proteins had been found in injured and naive axons of cortical neurons, respectively [9] . To confirm their axonal localization in DRGs, we collected total RNA from the axonal and cell body compartments of DRGs neurons grown in microfluidic chambers and performed RT-PCR for TC10 , Exoc3 , H1f0 (negative control; the cell body restricted transcript of a histone [14] ) and β-actin (positive control for an axonally localized mRNA [30] ). All mRNAs were detected in the cell body-derived material, but only β-actin and TC10 mRNA were present in the developing DRG axons ( Fig. 4a ). Because Exoc3 mRNA was absent from the developing DRG axons, we focused for the remainder of our studies on TC10 . To further confirm the axonal localization of TC10 mRNA, we used quantitative real-time PCR on total RNA collected from the axonal and cell body compartments of DRG neurons grown in microfluidic chambers. Twenty-four hours before collecting the RNA, we transfected either scrambled or TC10 targeting siRNA in the axons. The RNAi pathway is functional in developing axons [31] , a fact that can be used to selectively knockdown axonally localized mRNAs using siRNA without affecting mRNAs localized to the dendrites or cell bodies [14] , [31] . Transfection of the scrambled siRNA did not alter the observed levels for TC10 in the axons or cell bodies, while TC10 siRNA significantly reduced the axonal but importantly not the cell body levels ( Fig. 4b ). Further, to examine the levels of TC10 mRNA in axons relative to that of a more abundant mRNA like β-actin , we used digoxigenin-labelled riboprobes targeting TC10 or β-actin transcripts. Quantification of the FISH signal for either transcript revealed that TC10 mRNA is significantly less abundant than β-actin mRNA ( Fig. 4c ). In fact axonal TC10 mRNA is barely detectable by FISH in axons as had been seen before [32] , findings that parallel previous reports of very weak TC10 expression levels in uninjured motor neurons [8] and spinal cord and DRG neurons [33] . 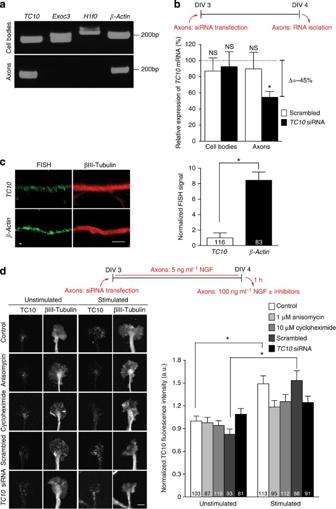Figure 4: TC10 is localized to axons of DRG neurons. (a) RT–PCR on total RNA purified from axons or cell bodies of DRG neurons grown in microfluidic chambers. All transcripts tested could be amplified from cell body RNA, while onlyTC10andβ-actinmRNAs were detected in the axonal material. The axonal mRNA preparation is not contaminated with cell body mRNA as seen by the absence ofH1f0. (b) Axons only were transfected with siRNA targetingTC10mRNA or a non-targeting, scrambled siRNA. Twenty-four hours laterTC10mRNA levels in axons and cell bodies were determined by real-time PCR. The axon-specific transfection ofTC10siRNA lead to a significant depletion ofTC10mRNA in axons but importantly did not affectTC10mRNA levels in the cell bodies. Data are mean±s.e.m. of 2−ΔCTvalues from three to four experiments. Dotted line indicates 2−ΔCTvalue forTC10mRNA in axons or cell bodies, respectively, of untransfected neurons. *P<0.01 (one sample t-test). (c) DRG neurons grown in microfluidic chambers were incubated with digoxigenin-labelled riboprobes directed againstTC10andβ-actin. FISH signal for a non-targetingGFPriboprobe was used to define non-specific background and was subtracted from the FISH signal forTC10andβ-actintranscripts in axons. Quantification of the FISH signal revealed a significantly lower level ofTC10mRNA in axons compared with that ofβ-actinmRNA. Scale bars, 5 μM. Data are mean±s.e.m. of FISH signal forTC10orβ-actinfrom three to four experiments. (d) Axons of DRG neurons grown in microfluidic chambers were stimulated with NGF for 10 min, and TC10 abundance was determined by quantitative immunofluorescence and normalized to growth cone area as defined by βIII-tubulin staining. Stimulation with NGF caused a significant increase in TC10 levels that was abolished by inhibition of local protein synthesis or axon-specificTC10knockdown. Data are mean±s.e.m. of the fluorescence intensity of TC10 immunostaining normalized to growth cone area from three individual experiments,nvalues represent the number of growth cones. *P<0.05 (one-way ANOVA). Scale bar, 5 μm. Figure 4: TC10 is localized to axons of DRG neurons. ( a ) RT–PCR on total RNA purified from axons or cell bodies of DRG neurons grown in microfluidic chambers. All transcripts tested could be amplified from cell body RNA, while only TC10 and β-actin mRNAs were detected in the axonal material. The axonal mRNA preparation is not contaminated with cell body mRNA as seen by the absence of H1f0 . ( b ) Axons only were transfected with siRNA targeting TC10 mRNA or a non-targeting, scrambled siRNA. Twenty-four hours later TC10 mRNA levels in axons and cell bodies were determined by real-time PCR. The axon-specific transfection of TC10 siRNA lead to a significant depletion of TC10 mRNA in axons but importantly did not affect TC10 mRNA levels in the cell bodies. Data are mean±s.e.m. of 2 −ΔC T values from three to four experiments. Dotted line indicates 2 −ΔC T value for TC10 mRNA in axons or cell bodies, respectively, of untransfected neurons. * P <0.01 (one sample t-test). ( c ) DRG neurons grown in microfluidic chambers were incubated with digoxigenin-labelled riboprobes directed against TC10 and β-actin . FISH signal for a non-targeting GFP riboprobe was used to define non-specific background and was subtracted from the FISH signal for TC10 and β-actin transcripts in axons. Quantification of the FISH signal revealed a significantly lower level of TC10 mRNA in axons compared with that of β-actin mRNA. Scale bars, 5 μM. Data are mean±s.e.m. of FISH signal for TC10 or β-actin from three to four experiments. ( d ) Axons of DRG neurons grown in microfluidic chambers were stimulated with NGF for 10 min, and TC10 abundance was determined by quantitative immunofluorescence and normalized to growth cone area as defined by βIII-tubulin staining. Stimulation with NGF caused a significant increase in TC10 levels that was abolished by inhibition of local protein synthesis or axon-specific TC10 knockdown. Data are mean±s.e.m. of the fluorescence intensity of TC10 immunostaining normalized to growth cone area from three individual experiments, n values represent the number of growth cones. * P <0.05 (one-way ANOVA). Scale bar, 5 μm. Full size image Next, we sought to confirm TC10 protein expression in growth cones and asked whether its level changed in response to treatment with NGF. TC10 was detectable at very low levels by immunofluorescence in distal axons and growth cones independent of stimulation with NGF, but a significant increase in TC10 levels after just 10 min of NGF stimulation was observed ( Fig. 4d ). Application of anisomycin or cycloheximide specifically to axons did not affect the level of TC10 protein in unstimulated axons and growth cones but reduced the NGF-dependent increase below the threshold for significance. Similarly, knockdown of axonal TC10 mRNA using siRNA did not alter baseline levels of TC10 but abolished the significant increase in response to NGF. Together these data establish that NGF-induced axonal elongation and membrane expansion are accompanied by intra-axonal TC10 synthesis. Local TC10 mRNA is required for axon outgrowth To determine whether axonally localized TC10 mRNA is required for NGF-induced axon outgrowth, we transfected scrambled or TC10 targeting siRNA specifically into axons of DRGs grown in microfluidic chambers and measured axon growth rates over a 1-h time period with and without NGF stimulation. Axonal growth rates for axons that were not transfected or received the non-targeting scrambled siRNA roughly doubled upon stimulation with NGF, as we had observed previously [14] ( Fig. 5a ). Growth rates in the absence of NGF stimulation were unchanged in axons transfected with TC10 siRNA compared with control axons. However, axons depleted of TC10 mRNA failed to increase their growth rate but rather stopped growing in response to NGF stimulation ( Fig. 5a ), indicating that axonal TC10 mRNA is not required for axon growth in general but specifically for increased outgrowth in response to NGF stimulation to support increased exocytosis of PPVs. The fact that axons lacking TC10 mRNA did not become insensitive to NGF treatment but rather reacted with growth arrest indicates the existence of parallel, NGF-dependent pathways that inhibit growth, as we have seen before in response to dominant negative disruption of PAR complex formation [14] . 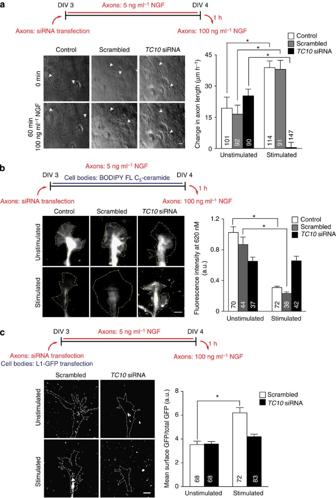Figure 5: Local synthesis of TC10 is required for axon growth and membrane expansion. Axons of DRG neurons grown in microfluidic chambers were transfected withTC10or scrambled siRNA. (a) Phase-contrast images of the same optical fields before and after stimulation with NGF for 1 h are shown with triangles indicating the measured terminal axonal segments. Knocking downTC10mRNA in the axonal compartment blocked the NGF-induced increase in axonal growth rates. Data are change in axonal length (mean±s.e.m.) from three to four independent experiments,nvalues listed represent the number of axons. *P<0.05 (one-way ANOVA). Scale bar, 10 μm. (b) Exocytosis of BODIPY FL C5-ceramide induced by stimulation of DRG axons with NGF was blocked upon depletion ofTC10mRNA in axons. The values for the unstimulated conditions are not significantly different. (c) Depletion ofTC10locally in axons abolished the significant increase in GFP-L1 at the growth cone surface following 1 h of treatment with NGF. Only growth cones showing above background GFP fluorescence intensities were included in the analysis. Data are mean±s.e.m. of the fluorescence intensities of individual growth cones from three independent experiments. *P<0.05 (one-way ANOVA). Scale bar, 5 μm. Figure 5: Local synthesis of TC10 is required for axon growth and membrane expansion. Axons of DRG neurons grown in microfluidic chambers were transfected with TC10 or scrambled siRNA. ( a ) Phase-contrast images of the same optical fields before and after stimulation with NGF for 1 h are shown with triangles indicating the measured terminal axonal segments. Knocking down TC10 mRNA in the axonal compartment blocked the NGF-induced increase in axonal growth rates. Data are change in axonal length (mean±s.e.m.) from three to four independent experiments, n values listed represent the number of axons. * P <0.05 (one-way ANOVA). Scale bar, 10 μm. ( b ) Exocytosis of BODIPY FL C 5 -ceramide induced by stimulation of DRG axons with NGF was blocked upon depletion of TC10 mRNA in axons. The values for the unstimulated conditions are not significantly different. ( c ) Depletion of TC10 locally in axons abolished the significant increase in GFP-L1 at the growth cone surface following 1 h of treatment with NGF. Only growth cones showing above background GFP fluorescence intensities were included in the analysis. Data are mean±s.e.m. of the fluorescence intensities of individual growth cones from three independent experiments. * P <0.05 (one-way ANOVA). Scale bar, 5 μm. Full size image Axonal TC10 synthesis is required for membrane expansion To determine whether the effect of axonal TC10 knockdown on outgrowth might be due to interference with the addition of phospholipids to the expanding plasma membrane, we repeated the two membrane exocytosis assays on axons transfected with scrambled or TC10 siRNA. Transfection with the scrambled siRNA did not have any effect, but axon-specific knockdown of TC10 mRNA completely abolished the increase in exocytosis in response to NGF as measured by BODIPY-ceramide dissipation ( Fig. 5b ). The difference between the red labelling in scrambled and TC10 siRNA transfected axons is statistically not significant but could indicate a minor contribution of local TC10 synthesis to exocytosis in unstimulated axons. We next investigated the effect of axonal TC10 mRNA knockdown on NGF-stimulated GFP-L1 translocation to the membrane ( Fig. 5c ). TC10 siRNA transfection did not change the amount of L1-GFP at the cell surface in the control condition but completely prevented the NGF-dependent increase in exocytosis, supporting the hypothesis that intra-axonal TC10 synthesis is required for exocytosis during stimulated axon outgrowth. Alternatively, the failure of axons to react to NGF upon knockdown of TC10 mRNA might be explained by reduced expression or exocytosis of the NGF receptor TrkA on the axonal surface rather than prevention of membrane expansion. To test for this possibility, we immunostained non-permeabilized axons and growth cones with an anti-TrkA antibody ( Fig. 6 ); no difference in surface TrkA expression was observed, clearly demonstrating that TC10 mRNA in axons is not required for the exocytosis of TrkA. Importantly, depletion of TC10 mRNA did not recapitulate the baseline effect seen before in the presence of protein synthesis inhibitors, confirming that axonal TC10 mRNA is required for exocytosis only under stimulated but not under basal conditions. 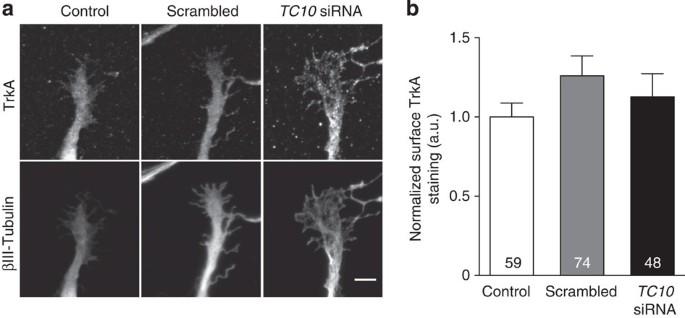Figure 6: TrkA surface expression does not require axonalTC10mRNA. (a) Axons of DRG neurons grown in microfluidic chambers were transfected withTC10or negative control siRNA. Depletion of axonalTC10mRNA does not interfere with TrkA trafficking to the cell surface; quantification in (b). Data are mean±s.e.m. of the fluorescence intensities of surface TrkA immunostaining from four individual experiments,nvalues listed represent the number of growth cones. Scale bar, 5 μm. Figure 6: TrkA surface expression does not require axonal TC10 mRNA. ( a ) Axons of DRG neurons grown in microfluidic chambers were transfected with TC10 or negative control siRNA. Depletion of axonal TC10 mRNA does not interfere with TrkA trafficking to the cell surface; quantification in ( b ). Data are mean±s.e.m. of the fluorescence intensities of surface TrkA immunostaining from four individual experiments, n values listed represent the number of growth cones. Scale bar, 5 μm. Full size image PI3K controls stimulated axon growth and membrane expansion So far, the results obtained in our study of the axonal role of TC10 mRNA are reminiscent of our previous data on the local translation of Par3 mRNA [14] : both mRNAs are axonally localized and their intra-axonal translation is required to support increased axonal growth rates in response to attractive factors but not for growth under baseline conditions. We therefore asked whether a common upstream regulator controls the intra-axonal translation of TC10 and Par3 . For example, PI3K activity is required for netrin-1-induced axonal mRNA translation in Xenopus retinal neuron axons [34] , as well as for exocytosis in growth cones in response to IGF-1 (ref. 35) [35] . Induction of intra-axonal Par3 and TC10 synthesis by PI3K could be a mechanism to spatially and temporally integrate cytoskeletal and membrane dynamics during stimulated axon growth. To investigate whether local PI3K signalling is required for increased axon outgrowth in response to NGF in DRG neurons, we performed an axon outgrowth assay as before in the presence of two PI3K inhibitors, wortmannin and LY294002. Axons of DRG neurons grown in microfluidic chambers were treated with NGF resulting in a significant increase in growth rate relative to vehicle that was completely inhibited by the selective application of wortmannin or LY294002 to axons ( Fig. 7a ). To determine whether the inhibition of NGF-induced axonal outgrowth was reflected by inhibition of membrane addition, we repeated the BODIPY-ceramide exocytosis assay in the presence of the PI3K inhibitors. Treatment of axons with wortmannin or LY294002 did not change the steady state levels of red labelling within growth cones indicating that PI3K activity is not required for exocytosis of PPVs in the absence of a stimulus ( Fig. 7b ). However, presence of either inhibitor completely prevented the dissipation of the red label upon NGF stimulation, demonstrating that PI3K activity is required for membrane addition during induced axon growth. 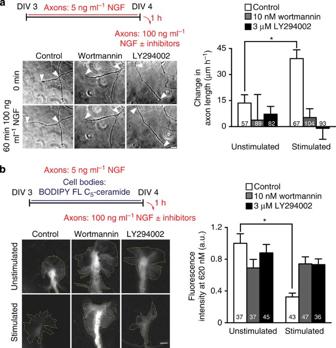Figure 7: Local PI3-kinase signaling controls axon outgrowth and membrane expansion. Axons of DRG neurons grown in microfluidic chambers were stimulated with NGF in the presence or absence of PI3K inhibitors. (a) NGF-stimulated increases in axon growth rates were inhibited by the PI3K inhibitors wortmannin (10 nM) or LY294002 (3 μM). Data are mean±s.e.m. growth rates from three independent experiments,nvalues listed represent the number of axons. *P<0.05 (one-way ANOVA). Scale bar, 10 μm. (b) Cell bodies of DRG neurons grown in microfluidic chambers were loaded with BODIPY FL C5 ceramide. After 24 h, axons were stimulated with NGF in the presence of PI3K inhibitors. Both inhibitors blocked the increase in NGF-stimulated exocytosis. Data are mean±s.e.m. of the fluorescence intensities of individual growth cones from three to four independent experiments. *P<0.05 (one-way ANOVA). Scale bar, 5 μm. Figure 7: Local PI3-kinase signaling controls axon outgrowth and membrane expansion. Axons of DRG neurons grown in microfluidic chambers were stimulated with NGF in the presence or absence of PI3K inhibitors. ( a ) NGF-stimulated increases in axon growth rates were inhibited by the PI3K inhibitors wortmannin (10 nM) or LY294002 (3 μM). Data are mean±s.e.m. growth rates from three independent experiments, n values listed represent the number of axons. * P <0.05 (one-way ANOVA). Scale bar, 10 μm. ( b ) Cell bodies of DRG neurons grown in microfluidic chambers were loaded with BODIPY FL C5 ceramide. After 24 h, axons were stimulated with NGF in the presence of PI3K inhibitors. Both inhibitors blocked the increase in NGF-stimulated exocytosis. Data are mean±s.e.m. of the fluorescence intensities of individual growth cones from three to four independent experiments. * P <0.05 (one-way ANOVA). Scale bar, 5 μm. Full size image PI3K-Rheb-mTOR signalling regulates TC10 and Par3 translation To directly test whether the intra-axonal synthesis of TC10 and Par3 is downstream of PI3K activity, we performed quantitative immunofluorescence on distal axons and growth cones treated with NGF in the presence of the PI3K inhibitor wortmannin. Treatment of DRG axons with NGF significantly increased Par3 protein levels in growth cones and distal axons within 10 min, consistent with previously published results [14] . Addition of wortmannin to the axons completely abolished the increase for both proteins without significantly altering their levels in growth cones not treated with NGF ( Fig. 8 ). PI3K activation can increase protein synthesis through activation of Akt causing the inhibition of TSC2 and consequently the activation of Rheb, which in turn activates mTOR [36] . Rheb activation of the mTOR-S6K-4EBP1 signalling pathway is farnesylation dependent [37] . To interfere with this pathway at multiple levels, we knocked down Rheb mRNA by transfecting siRNAs derived from published shRNA sequences [38] into the cell body compartment or applied the farnesyltransferase inhibitor FTI-277 (ref. 39) [39] and the mTOR inhibitor rapamycin [40] selectively to axons and repeated the TC10 and Par3 synthesis assays as before. Depletion of Rheb mRNA or presence of FTI-277 or rapamycin completely abolished the increase of both proteins’ abundances within growth cones in response to NGF treatment ( Fig. 8 ). From these findings emerges the model that the local activation of PI3K in response to attractive guidance cues triggers the Akt-Rheb-mTOR signalling pathway, resulting in the local translation of several transcripts leading in turn to the spatially and temporally coordinated activation of seemingly separate effector pathways in the control of axon outgrowth. 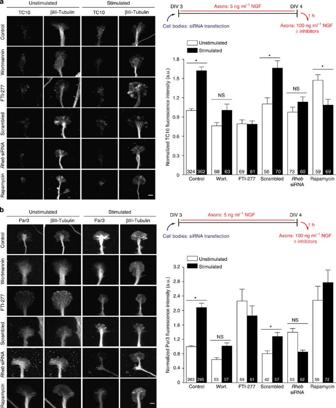Figure 8: NGF-stimulatedPar3translation occurs downstream of PI-3 kinase signalling. Axons of DRG neurons grown in microfluidic chambers were stimulated with NGF for 10 min in the presence or absence of a PI3K inhibitor, and changes in TC10 or Par3 protein levels were determined by quantitative immunofluorescence. Inhibition of PI3K (wortmannin), Rheb (FTI-277 or siRNA-mediated knockdown ofRhebmRNA in cell bodies) or mTOR (rapamycin) abolished the NGF-stimulated increases in TC10 (a) and Par3 (b) immunostaining levels within growth cones. Data are mean±s.e.m. of the fluorescence intensity of TC10 or Par3 immunostaining from three individual experiments,nvalues represent the number of growth cones. *P<0.05. Scale bar, 5 μm. Figure 8: NGF-stimulated Par3 translation occurs downstream of PI-3 kinase signalling. Axons of DRG neurons grown in microfluidic chambers were stimulated with NGF for 10 min in the presence or absence of a PI3K inhibitor, and changes in TC10 or Par3 protein levels were determined by quantitative immunofluorescence. Inhibition of PI3K (wortmannin), Rheb (FTI-277 or siRNA-mediated knockdown of Rheb mRNA in cell bodies) or mTOR (rapamycin) abolished the NGF-stimulated increases in TC10 ( a ) and Par3 ( b ) immunostaining levels within growth cones. Data are mean±s.e.m. of the fluorescence intensity of TC10 or Par3 immunostaining from three individual experiments, n values represent the number of growth cones. * P <0.05. Scale bar, 5 μm. Full size image Here we report a novel and unexpected mode for the locally restricted activation of exocyst-mediated secretion, the local synthesis of TC10. The exocyst is an evolutionarily conserved complex regulating the exocytosis or secretion of vesicles to target membranes. It functions in many diverse processes including cytokinesis, membrane growth, secretion of membrane proteins and autophagy [41] . Common to these functions is that the exocyst tethers the vesicles at precise locations at the cellular membrane, allowing fusion of the vesicles with the membrane. While we have found that the exocyst is regulated through local translation in a very specific context, NGF-stimulated axon outgrowth, it is possible that this mechanism is not unique to neurons. In fact, localized protein synthesis is not restricted to morphologically extremely polarized cells such as neurons but rather is a universally occurring phenomenon in many eukaryotic cells [42] . The best-studied function of the exocyst is its role in the insulin-dependent translocation of the glucose transporter GLUT4 in adipocytes [4] , [5] , a process that requires TC10 (ref. 4) [4] . Intriguingly, cycloheximide prevents insulin-induced increase of GLUT4 transporter surface expression in cultured rat adipocytes, and wortmannin inhibits the insulin induced but not the basal display of GLUT4 on the surface of these cells [43] . It is thus tempting to speculate that the signal-dependent local translation of TC10 downstream of PI3K is a general mechanism to localize the activity of the exocyst to specific domains of the cellular plasma membrane. TC10 mRNA levels are low in the nervous system compared with other Rho family members, especially RhoA, Rac and cdc42 (refs 8 , 33 ). A previous study reported 1.23 × higher cdc42 mRNA levels compared with TC10 in adult DRG axons, and TC10 but not cdc42 were below the threshold for present mRNA in embryonic DRG axons [32] . This is in line with several previously published mRNAs with well-described functions in developing axons, such as RhoA [10] , [31] , Par3 (ref. 14 ) or cofilin [12] , that were detected at very low levels or were even below the detection limit in microarray-based transcriptome analyses of embryonic DRG and Xenopus retinal ganglion cell axons [9] , [32] , [44] . Our data thus further exemplify the concept that the low abundance of an axonal mRNA cannot be used to deduce a lack of biological significance, especially as intra-axonal translation does not provide bulk material for the growing axons but rather fulfills a spatially restricted and temporally acute demand for greater protein levels within growth cones. Here we show that in developing DRG axons TC10 but not Exoc3 mRNA is present and required for induced membrane expansion and outgrowth. Previously, Exoc3 has been found to be increased (2.2-fold) in regenerating cortical mammalian axons while TC10 levels are reduced (0.6-fold). Together, these data suggest a difference in the local translatome during neurotrophin- and injury-induced axon extension. It remains an open question why different axonal growth modes would utilize two different axonally localized, exocyst-related mRNAs. We show that TC10 translation requires PI3K activity, and the same activity is required for NGF-induced axon growth in embryonic DRGs but not for regenerative growth in adult DRGs [45] . The presence of different mRNAs might be a reflection of the fact that developmental and regenerative axon growth are driven by different upstream regulators. Alternatively, axonal Exoc3 and TC10 mRNAs might subserve different functions in the regulation of membrane exocytosis. For example, in yeast the myosin V homologue, Myo2, interacts with the exocyst including Sec6p/Exoc3 (ref. 46) [46] . The presence of Exoc3 mRNA in regenerating axons might therefore be a reflection of increased transport of secretory vesicles, while local TC10 translation in developing axons triggers PPV tethering to specific secretion sites within the growth cones. Currently, it is unclear why some mRNAs are locally translated in developing axons. The majority of axonally localized proteins are synthesized in the cell body and transported into the cellular periphery, and even for proteins whose transcripts are axonally localized such as β-actin or β-tubulin the bulk of the axonal protein is cell body derived [47] . Further, local synthesis of many or even all proteins is not required for the growth of developing axons under baseline conditions but only in response to an external stimulus [10] , [14] , [47] , [48] . It is therefore important to ask which advantage the local synthesis of some proteins might have under these conditions compared with anterograde transport from the cell body. The results we present here and in a previous report [14] establish that two aspects of axon outgrowth, membrane expansion and cytoskeletal dynamics, are regulated through the intra-axonal synthesis of proteins that are pivotal in these cascades: Par3 and TC10. Our results thus provide evidence that intra-axonal translation can be a mechanism to ensure the spatially and temporally simultaneous activation of two seemingly unconnected pathways, such as cytoskeletal elongation and membrane expansion. These findings lead to the question whether the translation-activating signal downstream of PI3K acts on the individual mRNA species or on ribonucleoprotein (RNP) complexes in which transcripts coding for proteins with complementary function are copackaged. Association of RNA-binding proteins with discrete sets of mRNAs coding for functionally related proteins and coexistence of several mRNA species within shared RNP complexes have been unambiguously demonstrated in yeast [49] , [50] and are proposed to exist in eukaryotic cells [51] , [52] , [53] . It will be interesting to investigate whether the coordinated translation of TC10 and Par3 mRNAs downstream of PI3K activity is a reflection of the existence of these putative post-transcriptional RNA operons in axons and to establish whether other transcripts coding for proteins that function in induced axon elongation, like β-actin, are part of the same shared RNP complexes. Neuronal cell culture in microfluidic chambers All reagents were from Life Technologies (Carlsbad, CA) unless otherwise noted. DRGs were collected from Sprague–Dawley rat embryos (E15) of both sexes, dissociated with TrypLE and cultured in tripartite microfluidic chambers with two 200-μm-long microgrooves that allow the application of NGF, inhibitors or siRNA specifically to distal axons and growth cones without affecting the cell bodies [14] , [22] . All work involving animals was performed in accordance with the National Institutes of Health guidelines for the care and use of laboratory animals and was approved by The Animal Care and Use Committee of Columbia University. Microfluidic chambers were produced using masters replica molded from polyurethane plastic (Smooth Cast 310, Smooth-On, Easton, PA) [54] . (Poly)-dimethylsiloxane (PDMS) (Sylgard 184, Dow Corning, Midland, MI) was mixed (9 parts elastomer base to 1 part curing agent), degassed for 30 min, poured on the plastic masters and cured at 65 °C for longer than 4 h [55] . Individual microfluidic devices were cut from PDMS blocks with scalpels, and access ports were cut out using biopsy punches. The devices were cleaned using clean room tape, sterilized in 70% ethanol and air-dried before being mounted on cell culture dishes or glass coverslips coated with 100 μg ml −1 poly- L -lysine (Trevigen, Gaithersburg, MD). The growth medium (Neurobasal, 1x B27, 2 mM glutamate) was completely exchanged after 48 h. siRNA transfection in the axonal compartment was performed on DIV3, and all experiments were performed on DIV4. Quantification of membrane secretion Addition of new membrane within the growth cones was measured using two independent assays using BODIPY FL C 5 -ceramide or GFP-tagged L1, respectively. For the first assay, DRG explants were plated on poly- L -lysine coated coverslips. On DIV3, NGF concentration was reduced to 5 ng ml −1 . Twenty-four hours later, explants were incubated with the fluorescently labelled sphingomyelin and glucosylceramide precursor BODIPY FL C 5 -ceramide complexed to BSA in culture medium containing 5 ng ml −1 NGF. After incubation for 30 min at room temperature, the dye was removed and explants were washed once with culture medium. Fresh medium was added and explants were incubated at 37 °C for 3 h, followed by stimulation with 100 ng ml −1 NGF in the presence or absence of protein synthesis inhibitors (anisomycin, 1 μM or cycloheximide, 10 μM). One hour later, explants were washed once with PBS and fixed for 20 min in 4% paraformaldehyde (PFA) in PBS with 4% sucrose. BODIPY FL C 5 -ceramide in Golgi-derived vesicles was measured by the red fluorescence of the excimer. For examination of exocytosis in growth cones of axons in microfluidic chambers, a modification of the above protocol was used. On DIV3 BODIPY FL C 5 -ceramide was applied to the cell bodies of DRG neurons grown in microfluidic chambers (5 μM for 24 h), while medium in axonal compartments was exchanged with that containing 5 ng ml −1 . Twenty-four hours later axons were stimulated for 1 h with 100 ng ml −1 NGF in the presence of protein synthesis (anisomycin, 1 μM; cycloheximide, 10 μM or emetine, 2 μM) or PI3K inhibitors (LY294002, 3 μM or wortmannin, 10 nM). The neurons were fixed with 4% PFA in PBS/4% sucrose, washed and mounted. For the second assay, explants or dissociated DRG neurons were transfected with GFP -L1 (gift of Dr Galli, Paris, France) via the Sindbis-IRES system [10] , [14] , [31] , [56] . A modified Sindbis viral vector with reduced neuronal cytotoxicity due to the P76S point mutation in the nsP2 protein and containing an encephalomyocarditis virus internal ribosome entry site (IRES) was used together with the helper plasmid DH-BB (S. Schlesinger) to generate Sindbis pseudovirions according to the manufacturer’s instructions (Invitrogen). One day after transfection, neurons were treated with NGF (100 ng ml −1 ) or vehicle (0.1% BSA in PBS) for 1 h. Immediately after the treatment, live cultures were immunostained for surface GFP by incubation with antibodies to GFP (Abcam, Cambridge, MA; 1:50 dilution) in 3% BSA in PBS for 10 min at room temperature. Neurons were rinsed three times with 3% BSA in PBS and fixed for 15 min with 4% PFA, 4% sucrose. The fixative was quenched with 0.1 M glycine in PBS for 5 min, followed by three rinses with PBS. Cultures were then blocked in 10% BSA in PBS for 45 min at room temperature, followed by incubation with a secondary antibody to detect anti-GFP (Alexa 568 goat anti-chicken, Invitrogen, both 1:500 dilution) in 3% BSA in PBS, for 45 min at room temperature. Next, neurons were washed three times with PBS, rinsed one time by submersion in water and mounted with Prolong Gold antifade reagent. The GFP fluorescence did not distinguish between inter- and extracellular GFP and was used to outline the growth cones. The anti-GFP staining was specific for extracellular GFP. Images were quantified by dividing the average fluorescence of the secondary antibody labelling by the average fluorescence intensity of the GFP-L1 expression. Endocytosis assay Axons of DRG neurons grown in microfluidic chambers were transfected with siRNA against TC10 or negative control siRNA on DIV3. After 24 h, axons were incubated with 10 μM FM1-43FX dye in the presence or absence of protein synthesis inhibitors for 20 min. Neurons were then fixed with 4% PFA in PBS, washed and mounted. Z -stacks of images were acquired and fluorescence intensity of growth cones at 620 nM was quantified using ImageJ [57] . Detection of axonal mRNA For isolation of pure axonal RNA, E15 DRG neurons (60,000) were grown in tripartite microfluidic chambers. On DIV5, RNA was purified from distal axons or cell bodies using the PrepEase RNA Spin Kit (Affymetrix, INC, Santa Clara, CA) and further concentrated using the RNeasy MinElute Cleanup Kit (Qiagen, Valencia, CA). Purified total RNA was eluted in 10 μl nuclease-free water and was reverse transcribed to cDNA using the High Capacity cDNA Reverse Transcription Kit according to the manufacturer’s instructions (Life Technologies, Carlsbad, CA). cDNA was amplified using Phusion Taq DNA polymerase (Thermo Fisher Scientific, Waltham, MA) in 20 μl reactions: 2 μl cDNA, 10 μl 2 × master mix, 0.5 μM primers and 6 μl nuclease-free water. The protocol used was 98 °C for 10 s, 35 cycles: 98 °C for 1 s, 65 °C for 5 s, 72 °C for 15 s, 72 °C for 1 min. The following oligonucleotides were used as primers in the reaction: β-actin , 5′-AGCCATGTACGTAGCCATCC-3′ and 5′-CTCTCAGCTGTGGTGGTGAA-3′, TC10 , 5′-GTGGCCAAGGAAACTGTCAT-3′ and 5′-TGTGGCTTCAGATGCTGTTC-3′, ExoC3 , 5′-AAATGTTTGCCGTCTTGGAC-3′ and 5′-CTCAAGGCCTGGTGGTACAT-3′, H1f0 , 5′-GGGGTTGTGGGGGAGAAGAGGATAA-3′ and 5′-CAGGAAGAGGGGAAAGGAAACGAACA-3′. Two microlitres of the PCR product was further amplified using the same protocol and upstream primers as above and the following downstream primers: β-actin , 5′-ACGCTCGGTCAGGATCTTC-3′; TC10 , 5′-GCTGCCGCTTAGACCTTTAT-3′; Exoc3 , 5′-CACTGCACCAGCAGGTTCTT-3′; H1f0 , 5′-TAGGCACACTGAGGCACTTG-3′. For relative quantification of TC10 and β-actin , RNA was purified and reverse transcribed as above. cDNA was amplified in a reaction volume of 20 μl using 2 μl cDNA, 10 μl TaqMan gene expression master mix, 1 μl predesigned TaqMan probe and primers (Life Technologies assay IDs Rn00467435_m1 and Rn00667869_m1 for TC10 and β-actin , respectively). The amplification protocol used was 50 °C for 2 min, 95 °C for 10 min, 40 cycles: 95 °C for 15 s, 60 °C for 1 min. Fluorescence in situ hybridization Antisense riboprobes were transcribed in vitro from sense oligonucleotides containing a T7 promoter site (5′-GCCCTATAGTGAGTCGTATTAC-3′) at their 3′ end using the MEGAshortscript Transcription Kit (Life Technologies, Carlsbad, CA) and digoxigenin-conjugated UTP (Roche, Indianapolis, IN). A mix of five non-overlapping riboprobes with matching GC content was used to detect each mRNA. TC10.1: 5′-CTCACGGGCCCGGCGCGCTGATGCTCAAGTGCGTGGTGGTCGGCGACGGG-3′ TC10.2: 5′-AATGGGTACCAGAACTAAAGGAATATGCACCAAATGTCCCCTTCTTGTTA-3′ TC10.3: 5′-TAGCAAGACTGAATGACATGAAAGAAAAACCTGTCTGTGTGGAACAAGGA-3′ TC10.4: 5′-AGCAAAAGAGATCGGCGCATGCTGCTATGTGGAATGCTCAGCTCTGAC-3′ TC10.5: 5′-AAGGGTTTGAAGACTGTGTTTGACGAGGCTATCATAGCCATTTTAACT-3′ GFP.1: 5′-GATGCCACCTACGGCAAGCTGACCCTGAAGTTCATCTGCACCACCGGCAAG-3′ GFP.2: 5′-GACCACATGAAGCAGCACGACTTCTTCAAGTCCGCCATGCCCGAAGGCTAG-3′ GFP.3: 5′-ACTTCAAGGAGGACGGCAACATCCTGGGGCACAAGCTGGAGTACAACTACG-3′ GFP.4: 5′-AAGCAGAAGAACGGCATCAAGGTGAACTTCAAGATCCGCCACAACATCGAG-3′ GFP.5: 5′-AGTTCGTGACCGCCGCCGGGATCACTCTCGGCATGGACGAGCTGTACAAGG-3′ β-actin.1: 5′-TGAAGTACCCCATTGAACACGGCATTGTCACCAACTGGGACGATATGGAG-3′ β-actin.2: 5′-CCCTCTGAACCCTAAGGCCAACCGTGAAAAGATGACCCAGATCATGTTTG-3′ β-actin.3: 5′-CTACAGCTTCACCACCACAGCTGAGAGGGAAATCGTGCGTGACATTAAAG-3′ β-actin.4: 5′-TGACGTTGACATCCGTAAAGACCTCTATGCCAACACAGTGCTGTCTGGTG-3′ β-actin.5: 5′-GCACCATGAAGATCAAGATCATTGCTCCTCCTGAGCGCAAGTACTCTGTG-3′ Fluorescence in situ hybridization was performed as previously described [14] , [58] . Neurons grown in microfluidic chambers were fixed in 4% PFA in PBS for 20 min at room temperature. Following three washes with PBS, the cells were permeabilized with 0.5% Triton X-100 in PBS and washed twice with PBS. For hybridization, coverslips were incubated with a total of 100 ng digoxigenin-labelled riboprobe (20 ng of each of five riboprobes) in 30 μl hybridization buffer (50% formamide, 2 × SSC, 0.2% BSA, 1 mg ml −1 E. coli tRNA, 1 mg ml −1 salmon sperm DNA) overnight at 37 °C. The next day, coverslips were washed with constant agitation at 37 °C first with 50% formamide in 2 × SSC for 30 min followed by 50% formamide in 1 × SSC for another 30 min. Additional three washes for 15 min each were done at room temperature with 1 × SSC. The coverslips were washed three times for 5 min each with PBS containing 0.1% Tween-20, blocked with 3% BSA in PBST for 30 min and incubated with anti-digoxin (1:500; DI-22, Sigma) and anti β-III tubulin antibodies in blocking solution overnight at 4 °C. The coverslips were washed three times with PBST and incubated with secondary antibodies, Alexa 488 anti-mouse and 568 anti-chicken, for 1 h at room temperature, washed and mounted. Stacks of images of axons were acquired, and images were analysed using ImageJ. β-III tubulin staining was used to generate a mask within which the intensity of the FISH signal was quantified. Average fluorescence intensity of axonal fields that were incubated with a GFP probe was subtracted from the fluorescence intensities resulting from hybridization with TC10 or β-actin riboprobes. Immunofluorescence Axons of neurons grown in microfluidic chambers were stimulated with 100 ng ml −1 NGF for 10 min in the presence or absence inhibitors (cycloheximide, 10 μM; anisomycin, 1 μM; wortmannin, 10 nM; FTI-277, 100 nM; rapamycin, 10 nM). The neurons were fixed with 4% PFA in PBS/4% sucrose for 20 min at room temperature. The coverslips were washed three times in PBS and then blocked for 1 h with BGT buffer (3% BSA, 0.25% triton X-100 and 100 mM glycine) and then incubated with primary antibodies against TC10 (1:1,000, Abcam), Par3 (1:10,000, Millipore) and β-III tubulin (1:1,000, Abcam). Alexa 488 and 594 conjugated secondary antibodies were used at 1:500 dilutions. Z -stacks of images of growth cones were acquired. For quantification of surface expression of TrkA, medium in axonal compartments was exchanged with 5 ng ml −1 NGF on DIV 3 and transfected with siRNA against TC10 or negative control siRNA. The next day, axons were stimulated with 100 ng ml −1 for 1 h and then incubated with an anti-TrkA antibody (1:100, Abcam) for 10 min. Antibody was washed off with PBS, and neurons were fixed with 4% PFA in PBS for 20 min, permeabilized and blocked for 1 h with BGT buffer, followed by overnight incubation with an anti-β-III tubulin antibody. Alexa 488 and 594 secondary antibodies were used as already described. Stacks of images of growth cones were acquired, and intensity of surface TrkA immunostaining was measured using ImageJ. siRNA transfection Silencing of TC10 or Par3 mRNA was achieved by transfecting axons with siRNA using Neuroporter as the transfecting reagent (Genlantis, San Diego, CA) according to the manufacturer’s instructions. The following siRNAs were used to target TC10 (Genbank Accession Number NM_053522.1): 5′-GCAAGACUGAAUGACAUGA-3′ and 5′-GGAGGAAUGGGUACCAGAA-3′, Par3 [14] (NM_031235.1): 5′-CUGAAGAAAUCCAGCUCUU-3′ and 5′-CCUUAUCAAACCACAAGUG-3′, and Rheb [38] (NM_013216) 5′-AAUGGUUAUAUUCUUGUGU-3′ and 5′-GGGGCUGACCAGGCUACCA-3′. Negative control RNA was purchased from Life Technologies (Silencer Select Negative Control No. 1 siRNA). Axon outgrowth assay On DIV3, DRG neurons grown in microfluidic chambers were cultured in 5 ng ml −1 NGF, and axons were transfected with siRNA targeting TC10 or negative control RNA. After 24 h, phase-contrast images of the same axonal fields were acquired at 0 and 60 min after addition of 100 ng ml −1 NGF to axonal compartments. To examine the effect of phosphoinositide 3-kinase (PI3K) inhibitors on neurite growth, medium in axonal compartments was exchanged with 5 ng ml −1 NGF on DIV 3 and to 100 ng ml −1 NGF with PI3K inhibitors for 1 h on DIV4. As before, phase-contrast images were obtained at 0 and 60 min after addition of drugs. The length of axons within each treatment group before exposure to NGF was subtracted from the length measured after stimulation for 1 h and reported as change in length. Statistical analyses One-way ANOVA with Tukey’s post test was used for the comparison of three or more groups. Error bars represent mean±s.e.m. from a minimum of three independent biological replicate experiments. How to cite this article: Gracias, N. G. et al. Local translation of TC10 is required for membrane expansion during axon outgrowth. Nat. Commun. 5:3506 doi: 10.1038/ncomms4506 (2014). Disclaimer The content is solely the responsibility of the authors and does not necessarily represent the official views of the National Institutes of Health.